Observation of dark states in a superconductor diamond quantum hybrid system The hybridization of distinct quantum systems has opened new avenues to exploit the best properties of these individual systems. Superconducting circuits and electron spin ensembles are one such example. Strong coupling and the coherent transfer and storage of quantum information has been achieved with nitrogen vacancy centres in diamond. Recently, we have observed a remarkably sharp resonance (~1 MHz) at 2.878 GHz in the spectrum of flux qubit negatively charged nitrogen vacancy diamond hybrid quantum system under zero external magnetic field. This width is much narrower than that of both the flux qubit and spin ensemble. Here we show that this resonance is evidence of a collective dark state in the ensemble, which is coherently driven by the superposition of clockwise and counter-clockwise macroscopic persistent supercurrents flowing in the flux qubit. The collective dark state is a unique physical system and could provide a long-lived quantum memory. The last decade has seen that our understanding of the principles of quantum mechanics lead to the development of technologies underpinned by it. We are at the stage where real engineering of quantum devices is taking place. Hybridization of distinct quantum systems allows us to exploit the best properties of these individual systems without their weaknesses (refs 1 , 2 , 3 and references within). One well-known example of such hybridized quantum systems are superconducting circuits [4] , [5] coupled to electron spin ensembles [6] , [7] , [8] . These hybridized systems [9] , [10] , [11] , [12] , [13] , [14] , [15] , [16] , [17] , [18] , [19] , [20] , [21] have seen many fundamental experiments taking place including for instance, the strong coupling and the coherent transfer and storage of quantum information between the superconducting circuit and an electron spin ensemble from nitrogen vacancy (NV) centres in diamond [13] , [14] , [15] , [16] , [17] . In these experiments, the negatively charged nitrogen vacancy (NV − ) centres were generally considered as an ensemble of two-level systems where one mode of the ensemble collectively coupled to the superconducting circuit. However, the ground-state manifold of the NV − centre is in fact a three-level system, which could show phenomena beyond those available in two-levels systems. Dark states are a particular state of a three-level atom or molecule driven by two fields, which cannot absorb or emit photons [22] , [23] . Further, dark states are not solely the province of single atoms but can be seen in ensembles of atoms as well. While such effects have generally been investigated in quantum optical systems [24] , [25] , [26] , [27] , the potential exists from them to be observed in hybrid solid-state systems. Here we are going to consider a hybrid system ( Fig. 1 ) composed of an ensemble of NV − centres coupled with a gap-tuneable flux qubit [28] , [29] . The gap-tuneable flux qubit can be considered as a strongly coupled coherent source of single microwave photons that can be used to pump the NV − centre ensemble. Depending on whether an external magnetic field is applied to split these two upper levels or not, the microwave photon can be absorbed by either of the upper levels or at zero external field by a coherent superposition of those levels. Next, a strain coupling between these two upper levels allows exchange of excitations in these levels and so is also a form of effective driving term. Having these two fields opens up the possibility for the observation of a collective dark state. A number of recent experiments [13] , [16] have hinted at a fine spectroscopy feature near the 2.878-GHz resonance but these have not been really explored. In this work we investigate its nature. 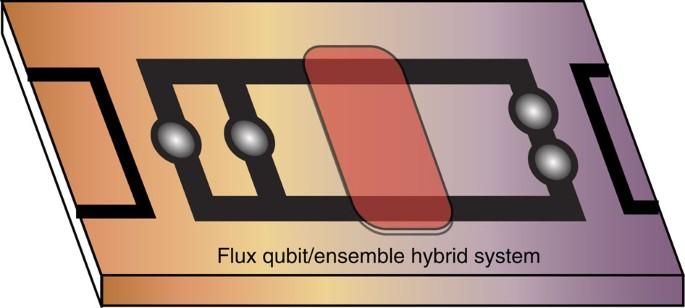Figure 1:Illustration of a hybrid-coupled system. The hybrid system is composed of a gap-tuneable flux qubit and an ensemble of NV−centres in diamond. The flux qubit is composed of four junctions (represented by the shaded circles). Input lines to adjust and drive the qubit are shown coming from the edges. The ensemble (light red coloured object) sits on top of the qubit. Figure 1: Illustration of a hybrid-coupled system . The hybrid system is composed of a gap-tuneable flux qubit and an ensemble of NV − centres in diamond. The flux qubit is composed of four junctions (represented by the shaded circles). Input lines to adjust and drive the qubit are shown coming from the edges. The ensemble (light red coloured object) sits on top of the qubit. Full size image Characterization Our characterization of this hybrid system [16] begins with spectroscopic measurements (shown in Fig. 2 ) of two physically different ensembles (A and B) with NV − density of ~4.7 × 10 17 cm −3 and 1.1 × 10 18 cm −3 , respectively. Both our samples ( Fig. 2a,c ) show significant hybridization near the optimal point , clearly indicating strong coupling. The splitting between the hybridized peaks is 28 MHz and 42 MHz, respectively. The energy spectrum shows a narrow peak located in the middle of the avoid crossing structure ( Fig. 2a,c ). To highlight this narrowness further, we show in Fig. 2d a fine scan of the spectrum (c) near the centre peak. The narrowest full width at half maximum of the peak is about 1.0 MHz ( Fig. 2b ) and 2.2 MHz ( Fig. 2e ), respectively. This line width is much narrower than the flux qubit or ensembles natural line widths. 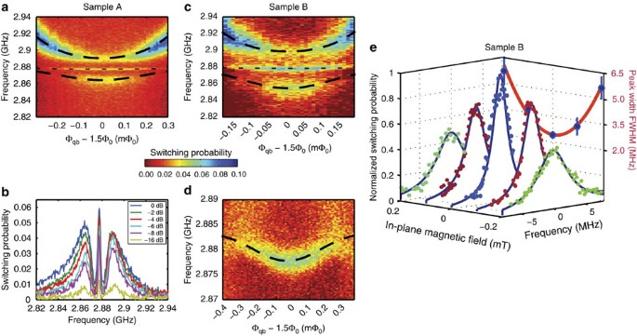Figure 2: Spectroscopy characterization of the hybrid system. Energy spectrum of a gap-tuneable flux qubit coupled separately to two different density NV−spin ensembles (samples A and B), the first having 4.7 × 1017cm−3(a,b) and the second 1.1 × 1018cm−3(c–e). The peak splittings were determined as 28 MHz for sample A and 42 MHz for sample B. Both spectroscopic measurementsaandcshow a sharp peak located in the middle of the avoided crossing structure. Inbwe show the microwave power dependence of the spectrum for a fixed flux bias (Φqb=1.5 Φ0). The centre sharp peak exists for all probe powers and shows a higher amplitude than the outer two broader peaks implying it is unlikely to result from a two-photon/nonlinear process. At the pump power used, our flux qubit would normally show power-broadening effects. Ind, a fine scan of the spectrum (c) near the centre peak part is illustrated. The sharp peak shows a small flux bias Φqbdependence (Φqbis the flux through the qubit loop). The eigen energies (black dashed lines) of the spectrumsa,canddcan be reproduced by diagonalizing the full Hamiltonian of the system (Supplementary Note 1). Ine, the normalized switching probability of the central peak is shown for several small in-plane magnetic fields (our diamond crystal was attached on top of the superconducting circuit with the (001) surface facing the flux qubit). The small in-plane magnetic field splits the degenerate excited states |±1› of the NV−ensemble weakening the effect of the strain interaction. The larger the splitting, the weaker the interaction. The full width at half maximum of the peak is minimal at zero in-plane magnetic field and becomes larger when the amplitude of the magnetic field increases. Spectraaandbwere measured with a 0-mT in-plane magnetic field whilecanddwere measured with a small −0.1 mT in-plane magnetic field. The error bars represent the 95% confidence interval while fitting to the resonance peaks. Figure 2: Spectroscopy characterization of the hybrid system. Energy spectrum of a gap-tuneable flux qubit coupled separately to two different density NV − spin ensembles (samples A and B), the first having 4.7 × 10 17 cm −3 ( a , b ) and the second 1.1 × 10 18 cm −3 ( c – e ). The peak splittings were determined as 28 MHz for sample A and 42 MHz for sample B. Both spectroscopic measurements a and c show a sharp peak located in the middle of the avoided crossing structure. In b we show the microwave power dependence of the spectrum for a fixed flux bias (Φ qb =1.5 Φ 0 ). The centre sharp peak exists for all probe powers and shows a higher amplitude than the outer two broader peaks implying it is unlikely to result from a two-photon/nonlinear process. At the pump power used, our flux qubit would normally show power-broadening effects. In d , a fine scan of the spectrum ( c ) near the centre peak part is illustrated. The sharp peak shows a small flux bias Φ qb dependence (Φ qb is the flux through the qubit loop). The eigen energies (black dashed lines) of the spectrums a , c and d can be reproduced by diagonalizing the full Hamiltonian of the system ( Supplementary Note 1 ). In e , the normalized switching probability of the central peak is shown for several small in-plane magnetic fields (our diamond crystal was attached on top of the superconducting circuit with the (001) surface facing the flux qubit). The small in-plane magnetic field splits the degenerate excited states |±1› of the NV − ensemble weakening the effect of the strain interaction. The larger the splitting, the weaker the interaction. The full width at half maximum of the peak is minimal at zero in-plane magnetic field and becomes larger when the amplitude of the magnetic field increases. Spectra a and b were measured with a 0-mT in-plane magnetic field while c and d were measured with a small −0.1 mT in-plane magnetic field. The error bars represent the 95% confidence interval while fitting to the resonance peaks. Full size image The model To establish the mechanism causing this narrow central peak, we need to consider a Hamiltonian model of a driven flux qubit coupled to an ensemble of NV − centres. The full description is presented in Supplementary Note 1 , but this can be significantly simplified when we consider that our flux qubit will only drive a few excitations in the ensemble. In such a situation we can model the spin ensemble as a number of harmonic oscillators [30] , [31] , [32] and so write the Hamiltonian after a rotating wave approximation as where σ ± are the raising/lowering operators of the flux qubit in the energy basis |0› qb and |1› qb , Δ represents the flux qubit’s tunnel energy splitting while ε is its energy bias. The ensembles are represented as two harmonic oscillators and where and with . GHz is the mean zero-field splitting between the lowest energy level of the NV − centres and the two excited states. The term couples the two harmonic oscillators together allowing exchange of excitations between them. It is in effect a direct current (DC) driving term whose magnitude can be varied by detuning the and harmonic oscillators energy levels. The term J arises from both strain and Zeeman effects. The flux qubit couples only to one mode of this ensemble, which we describe by . It represents the flux qubit driving the ensemble with a single excitation. The coupling strength G of this interaction is given by , where N is the number of centres in the coupled ensemble, g e μ B /2 π =28 MHz mT −1 and is the perpendicular component to the NV axis of the magnetic field generated by the flux qubit. This coupling strength can be tuned by moving the flux qubit off-resonance with the ensemble (non-zero ε ). Energy levels and their associated states Tuning the energy gap of the flux qubit (Δ) to D , we can straightforwardly determine the eigen energies and eigenstates of the hybrid system using equation (1). We choose for simplicity θ = π /2 to illustrate this (in Supplementary Note 1 , we relax this constraint). The eigen energies are plotted against J in Fig. 3a . The lowest energy level labelled by L0 corresponds to the ground state |0› qb |0› ens where . 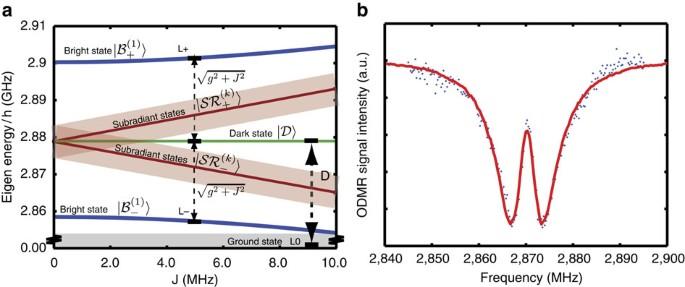Figure 3: Energy-level diagram of the coupled system. Ina, we illustrate the energy-level diagram for the superconducting flux qubit—NV−centre ensemble as a function of theJat the optimal point Φqb=1.5Φ0. The energy levels for the bright states are labelled bywhile the dark stateenergy is seen at 2.878 GHz. There are many subradiant statesthat can be broadened significantly by strain variation and inhomogenous broadening (light red). Inb, the optically detected magnetic resonance spectrum of the NV−ensemble is given (at room temperature). The two excited states at thekth spin wave are energetically separated byJ. The blue dots denotes the experimentally measured data while the red line shows our numerically simulated results (described inSupplementary Note 2). With the room temperature measurementwhile at the low temperature the zero-field splitting increases to(refs13,16,36). The energy level L−(L+) corresponds to the single-excitation dressed bright states Figure 3: Energy-level diagram of the coupled system. In a , we illustrate the energy-level diagram for the superconducting flux qubit—NV − centre ensemble as a function of the J at the optimal point Φ qb =1.5Φ 0 . The energy levels for the bright states are labelled by while the dark state energy is seen at 2.878 GHz. There are many subradiant states that can be broadened significantly by strain variation and inhomogenous broadening (light red). In b , the optically detected magnetic resonance spectrum of the NV − ensemble is given (at room temperature). The two excited states at the k th spin wave are energetically separated by J . The blue dots denotes the experimentally measured data while the red line shows our numerically simulated results (described in Supplementary Note 2 ). With the room temperature measurement while at the low temperature the zero-field splitting increases to (refs 13 , 16 , 36 ). Full size image The transitions between corresponds to the two broader peaks shown in Fig. 2a,c near . These transitions are being directly driven. Next in our diagram are energy levels associated with the subradiant states. These are composed of states having only a single excitation in the ensemble. These states have no |1› qb |0› ens component and so cannot be detected using flux qubit spectroscopic measurements. For finite J , these subradiant states are split either above or below the 2.878-GHz resonance ( Fig. 3a ) and in the limit be written as the spin waves ( k >0) with an energy of . These spin waves are orthogonal to the k =0 mode and so do not couple to the flux qubit. Finally, in terms of single excitation energy levels is the eigenstate at 2.878 GHz, which corresponds to This state can further be written in the form where . The form of dark state | › is important because it contains both components of an excitation in the flux qubit |1› qb |0› ens and the ensemble. The component |1› qb |0› ens implies that a signal will be seen at 2.878 GHz in the spectroscopic measurements (observed in Fig. 2 ). Next, as we tune the flux qubit away from the resonance point using the energy bias ε , we would expect to see a slight quadratic Φ qb dependence in the observed resonance frequency ( Fig. 2d ) owing to the small |1› qb |0› ens component in | ›. When we apply an in-plane magnetic field, we effectively strengthen the driving field J and so we increase the contribution of the |1› qb |0› ens component to . The population of this component is proportional to J and so we should expect to observe a quadratic dependance in the observed line width (observed in Fig. 2e ). We can also understand the power-dependent measurements in ( Fig. 2b ). Given that the J field is not changing during these experiments, we would expect the area of the central peak to decrease at approximately the same linear rate as the outer broader peaks as the pump field driving the flux qubit decreases. This is clearly what is seen even at very low pump powers ( Fig. 4 ) and clearly shows this is not a two-photon process. The amplitude of the centre peak being higher than the outer peaks is also an indicator. 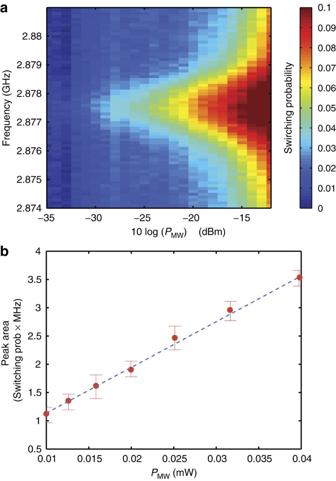Figure 4: Power dependence of the central peak of sample A. Ina, we show the energy spectrum of the gap-tuneable flux qubit coupled separately the NV−spin ensemble for varying microwave pump powerPMV(mW) at room temperature. Inb, the area of the central peak is shown againstPMV(mW). The error bars represent the 95% confidence interval while fitting to the resonance peaks. The dashed line represents a simple linear fit to the data points. Figure 4: Power dependence of the central peak of sample A. In a , we show the energy spectrum of the gap-tuneable flux qubit coupled separately the NV − spin ensemble for varying microwave pump power P MV (mW) at room temperature. In b , the area of the central peak is shown against P MV (mW). The error bars represent the 95% confidence interval while fitting to the resonance peaks. The dashed line represents a simple linear fit to the data points. Full size image Coherence properties The line width of these peaks depends on the coherence properties of our hybrid system. Surprisingly, the line width of the central peak, 1.0 MHz for sample A and 2.2 MHz for sample B, seems quite narrow compared with the usual coherence properties of the system. The measured flux qubit coherence properties at the optimal point are (relaxation), (dephasing) [16] . However, in the spectroscopic measurements, power broadening of makes these much worse. Further, the coherence properties also decrease rapidly as we move away from the optimal point. As is mainly composed of the state , it is now easy to understand why the dark states’ line width does not change much as the flux qubit moves away from the optimal point (by increasing ε ). Although the flux qubit line width increases, it has a minimal contribution to (proportionally to J 2 /( G 2 + J 2 )). Next, the electron spin ensemble T 1 (NV) has been measured to be (ref. 15 ); however, is much shorter (tens of nanoseconds) in our case [17] . Inhomogenous broadening due to random magnetic fields caused by nitrogen (P1) and other centres in the diamond sample A (B) is likely to be the primary cause of this and it has been derived from the fitting to the spectrum data at ~3.1 MHz (7.8 MHz; see Supplementary Notes 1 and 2 ). The distribution of the strain field is ~4.4 MHz (7.6 MHz) while fluctuations in the zero-field splitting D are 0.45 MHz (0.75 MHz). An always-on hyperfine coupling to thermalized nitrogen nuclear spins is ~2.3 MHz (ref. 17 ). These values are consistent with the previous experimental results [16] , [17] . The measured line width of the central peak is narrower than all these (apart from D fluctuations). Our modelling of these system indicates that this central peaks is not limited by the effects of the strain field or inhomogenous broadening. Instead, it seems currently limited by qubit power broadening and zero-field fluctuations. The energy diagram in ( Fig. 3a ) illustrates why this collective state has such a narrow line width (and hence long lifetime). The state | › would couple with other subradiant states and dephase quickly if a significant number of them existed near 2.878 GHz. Fortunately, the existence of inhomogenous broadening and the strain field induces an energy shift from 2.878 GHz on the subradiant states leaving this collective dark state well isolated. Since the dephasing process is induced by low-frequency noise, such an energy gap can suppress unwanted transitions between ( ) and environmental states ( ). This is quite different from what happens with general atom-based dark states. We have simulated the effects of strain variation and inhomogenous broadening using the full Hamiltonian (detailed in Supplementary Note 1 ) along with decoherence on the flux qubit, enabling us to confirm our analytical results described above. Moreover, the room temperature optically detected magnetic resonance spectrum measurements [33] , [34] , [35] support our interpretation that our subradiant states’ energies are sparsely occupied near the central peak in Fig. 3b . At room temperature, this reduction in population is at 2.87 GHz but shifts to 2.878 GHz at mK temperatures [36] . Thus, we have strong evidence for the existence of this collective dark state. Generally with dark states, if one turns off the control field, the dark state disappears. In our situation, here we cannot turn off the DC J field but by applying a large magnetic field we can split the |±1› levels by nearly 100 MHz. The coupling field is then effectively off-resonance because of the energy splitting. Experimentally, only double peaks showing the hybridization are seen either resonant with the |0›↔|+1› transition or the |0›↔|−1› transition. No fine feature is seen at 2.878 GHz. This is further evidence of our collective dark state (in Supplementary Note 3 where we show how the observed phenomenon is inconsistent with an ensemble of two-level systems). To summarize, we have experimentally observed a narrow peak in the avoided crossing structure of the energy spectrum in the flux qubit NV − diamond hybrid system. Our analysis indicates that this is the signature of a collective dark state, which should be long lived and could provide an alternative approach for quantum memories. The lifetime of this peak can further be increased in the near future with higher quality diamond samples that possess a smaller number of nitrogen centres and that have reduced homogenous broadening and zero-field fluctuations. This can be partially achieved by using electron beam irradiation to form the NV − centres. Measurements Spectroscopic measurements were achieved by initializing the hybrid system in its ground state through relaxation. A 1-μs-long microwave pulse was applied to the flux qubit followed immediately by a current pulse to the DC-superconducting quantum interference device for detecting the state of the qubit. By repeating the measurement several thousand times, we obtain the switching probability P sw , which is proportional to the qubit excited-state population. How to cite this article: Zhu, X. et al. Observation of dark states in a superconductor diamond quantum hybrid system. Nat. Commun. 5:3524 doi: 10.1038/ncomms4524 (2014).